RETRACTED ARTICLE: Pericyte loss influences Alzheimer-like neurodegeneration in mice Pericytes are cells in the blood–brain barrier that degenerate in Alzheimer’s disease (AD), a neurological disorder associated with neurovascular dysfunction, abnormal elevation of amyloid β-peptide (Aβ), tau pathology and neuronal loss. Whether pericyte degeneration can influence AD-like neurodegeneration and contribute to disease pathogenesis remains, however, unknown. Here we show that in mice overexpressing Aβ-precursor protein, pericyte loss elevates brain Aβ40 and Aβ42 levels and accelerates amyloid angiopathy and cerebral β-amyloidosis by diminishing clearance of soluble Aβ40 and Aβ42 from brain interstitial fluid prior to Aβ deposition. We further show that pericyte deficiency leads to the development of tau pathology and an early neuronal loss that is normally absent in Aβ-precursor protein transgenic mice, resulting in cognitive decline. Our data suggest that pericytes control multiple steps of AD-like neurodegeneration pathogenic cascade in Aβ-precursor protein-overexpressing mice. Therefore, pericytes may represent a novel therapeutic target to modify disease progression in AD. Pericytes are vascular mural cells embedded within the basement membrane of blood microvessels, a site of the blood–brain barrier in vivo [1] . Pericytes are uniquely positioned within the neurovascular unit between endothelial cells of brain capillaries, astrocytes and neurons [2] . Recent studies have shown that pericytes regulate the key neurovascular functions including blood–brain barrier formation and maintenance, vascular stability and angioarchitecture, regulation of capillary blood flow, and clearance of toxic cellular byproducts necessary for normal functioning of the central nervous system [3] , [4] , [5] , [6] , [7] . Studies using adult viable pericyte-deficient mice have shown that pericyte loss leads to brain vascular damage by two parallel pathways. The first is blood–brain barrier breakdown associated with brain accumulation of serum proteins and several potentially toxic blood-derived products. The second is the reduction in brain microcirculation causing diminished brain capillary perfusion and tissue hypoxia, ultimately leading to secondary neuronal degenerative changes [3] , [5] , [7] , [8] . Neurovascular dysfunction [8] , [9] , [10] , microvascular reductions [2] , [8] , [9] , [10] and pericyte degeneration and loss [8] , [11] , [12] , [13] have been demonstrated in Alzheimer’s disease (AD), a neurodegenerative disorder associated with abnormal elevation of amyloid β-peptide (Aβ) [14] , [15] , [16] , tau pathology [17] , [18] and neuronal loss [14] , [15] , [16] , [17] , [18] . Whether pericyte loss can influence the natural course of AD-like neurodegeneration and contribute to disease pathogenesis and accumulation of AD pathology remains, however, unknown. To address this question, we crossed transgenic mice overexpressing the Swedish mutation of human Aβ-precursor protein ( APP sw/0 ) [19] with pericyte-deficient platelet-derived growth factor receptor-β ( Pdgfrβ +/− ) mice [4] , [5] . APP sw/0 mice develop Aβ elevation, amyloid plaques and correlative memory deficits but do not have significant tau pathology or neuronal loss [19] , [20] . Pdgfrβ +/− mice exhibit a moderate but age-dependent progressive loss of brain pericytes because of PDGFRβ deficiency in pericytes that disrupts normal endothelial-derived platelet-derived growth factor B (PDGF-BB) signal transduction to PDGFRβ, regulating pericyte proliferation, migration and recruitment to the vascular wall [4] , [5] . Here we show that pericyte loss in APP sw/0 mice elevates brain Aβ levels and accelerates amyloid angiopathy and cerebral β-amyloidosis by diminishing clearance of soluble Aβ from the brain interstitial fluid prior to Aβ deposition. We further show that pericyte deficiency leads to the development of tau pathology and an early neuronal loss that is normally absent in APP sw/0 mice, resulting in accelerated cognitive decline. Thus, pericyte loss has an effect on multiple steps of AD-like neurodegeneration pathogenic cascade in APP sw/0 mice suggesting that pericytes may represent a novel therapeutic target to modify disease progression in AD. Pericyte loss accelerates Aβ pathology in APP sw/0 mice APP sw/0 ; Pdgfrβ +/− mice exhibited an accelerated age-dependent loss of pericytes compared with either control APP sw/0 ; Pdgfrβ +/+ mice or Pdgfrβ +/− mice beginning at 1 month of age and reaching within 9 months a significant 55% loss compared with 17 and 26% pericyte losses found in APP sw/0 ; Pdgfrβ +/+ and Pdgfrβ +/− littermates, respectively ( Fig. 1a,b ). Compared with APP sw/0 ; Pdgfrβ +/+ mice, pericyte-deficient APP sw/0 ; Pdgfrβ +/− littermates developed robust A β pathology within 9 months of age including a twofold increase in total human Aβ40 and Aβ42 levels ( Fig. 2a,b ) and an accelerated development of cerebral amyloid angiopathy and parenchymal amyloid deposition, as illustrated in the cortex by multiphoton imaging of X04-positive amyloid [21] , indicating fivefold and threefold elevations in cerebral amyloid angiopathy and parenchymal amyloid load, respectively ( Fig. 2c–e ). Aβ load determined by immunostaining was also increased by five- to sixfold in the cortex and hippocampus of APP sw/0 ; Pdgfrβ +/− compared with APP sw/0 ; Pdgfrβ +/+ mice, respectively ( Fig. 2f–h ). 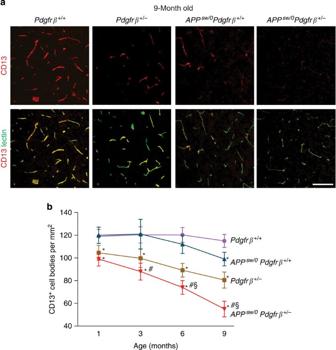Figure 1: Progressive degeneration of pericytes inAPPsw/0Pdgfrβ+/−mice. (a) Confocal microscopy analysis of CD13-positive pericytes and lectin-positive capillary endothelium in the cortex of 9-month-oldPdgfrβ+/+, Pdgfrβ+/−,APPsw/0;Pdgfrβ+/+andAPPsw/0;Pdgfrβ+/−mice. Scale bar, 100 μm. (b) Quantification of CD13-positive pericytes in the cortex and hippocampus of 1-, 3-, 6- and 9-month-oldPdgfrβ+/+, Pdgfrβ+/−,APPsw/0;Pdgfrβ+/+andAPPsw/0;Pdgfrβ+/−age-matched littermates. Mean±s.e.m.,n=6 mice per group. Data from the cortex and hippocampus were pooled because there were no significant differences between these two regions. *P<0.05, all other groups compared withPdgfrβ+/+;#P<0.05,APPsw/0;Pdgfrβ+/−compared withAPPsw/0;Pdgfrβ+/+;§P<0.05,APPsw/0;Pdgfrβ+/−compared withPdgfrβ+/−. All comparisons are by analysis of variance (ANOVA) followed by Tukey’spost-hoctests. Figure 1: Progressive degeneration of pericytes in APP sw/0 Pdgfrβ +/− mice. ( a ) Confocal microscopy analysis of CD13-positive pericytes and lectin-positive capillary endothelium in the cortex of 9-month-old Pdgfrβ +/+ , Pdgfrβ +/− , APP sw/0 ; Pdgfrβ +/+ and APP sw/0 ; Pdgfrβ +/− mice. Scale bar, 100 μm. ( b ) Quantification of CD13-positive pericytes in the cortex and hippocampus of 1-, 3-, 6- and 9-month-old Pdgfrβ +/+ , Pdgfrβ +/− , APP sw/0 ; Pdgfrβ +/+ and APP sw/0 ; Pdgfrβ +/− age-matched littermates. Mean±s.e.m., n =6 mice per group. Data from the cortex and hippocampus were pooled because there were no significant differences between these two regions. * P <0.05, all other groups compared with Pdgfrβ +/+ ; # P <0.05, APP sw/0 ; Pdgfrβ +/− compared with APP sw/0 ; Pdgfrβ +/+ ; § P <0.05, APP sw/0 ; Pdgfrβ +/− compared with Pdgfrβ +/− . All comparisons are by analysis of variance (ANOVA) followed by Tukey’s post-hoc tests. 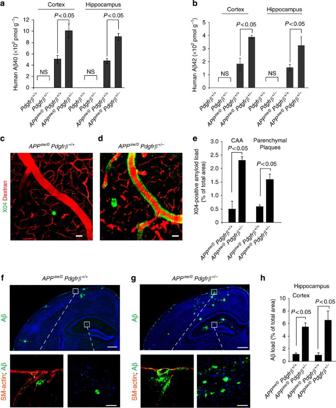Figure 2: Pericyte deficiency accelerates Aβ pathology inAPPsw/0Pdgfrβ+/−mice. (a–e) Human Aβ40 and Aβ42 levels in the cortex and hippocampus (a,b)in vivomultiphoton microscopy of cortical angiograms with Texas-Red-conjugated dextran (red) and methoxy-X04-positive amyloid (green) (c,d, scale bar, 50 μm) and quantification of cerebral amyloid angiopathy (CAA) and parenchymal methoxy-X04-positive amyloid (e) in 9-month-oldAPPsw/0;Pdgfrβ+/+andAPPsw/0;Pdgfrβ+/−littermates. Ina,b, human Aβ40 and Aβ42 levels were determined in 9-month-oldPdgfrβ+/+andPdgfrβ+/−mice. (f–h) Representative cortex and hippocampus sections stained with antibody against Aβ (6E10) (f,gupper panel scale bar, 400 μm; lower panel scale bar, 50 μm) and quantification of Aβ load (h) in 9-month-oldAPPsw/0;Pdgfrβ+/+andAPPsw/0;Pdgfrβ+/−mice. Insets inf,g: left, amyloid (green) and vascular smooth muscle cell actin (SM-actin, red) in the pial vessel on the surface of the brain; right, Aβ deposits in the hippocampus (green). In panelsa,b,e,h, values are means±s.e.m.,n=6 mice per group. Ina,b,P<0.05 by ANOVA followed by Tukey’spost-hoctests. NS, nonsignificant. Ine,h,P<0.05 by Student’st-test. Full size image Figure 2: Pericyte deficiency accelerates Aβ pathology in APP sw/0 Pdgfrβ +/− mice. ( a – e ) Human Aβ40 and Aβ42 levels in the cortex and hippocampus ( a , b ) in vivo multiphoton microscopy of cortical angiograms with Texas-Red-conjugated dextran (red) and methoxy-X04-positive amyloid (green) ( c , d , scale bar, 50 μm) and quantification of cerebral amyloid angiopathy (CAA) and parenchymal methoxy-X04-positive amyloid ( e ) in 9-month-old APP sw/0 ; Pdgfrβ +/+ and APP sw/0 ; Pdgfrβ +/− littermates. In a , b , human Aβ40 and Aβ42 levels were determined in 9-month-old Pdgfrβ +/+ and Pdgfrβ +/− mice. ( f – h ) Representative cortex and hippocampus sections stained with antibody against Aβ (6E10) ( f , g upper panel scale bar, 400 μm; lower panel scale bar, 50 μm) and quantification of Aβ load ( h ) in 9-month-old APP sw/0 ; Pdgfrβ +/+ and APP sw/0 ; Pdgfrβ +/− mice. Insets in f , g : left, amyloid (green) and vascular smooth muscle cell actin (SM-actin, red) in the pial vessel on the surface of the brain; right, Aβ deposits in the hippocampus (green). In panels a , b , e , h , values are means±s.e.m., n =6 mice per group. In a , b , P <0.05 by ANOVA followed by Tukey’s post-hoc tests. NS, nonsignificant. In e , h , P <0.05 by Student’s t -test. Full size image Surprisingly, loss of pericytes increased by 12- to 15-fold cortical and hippocampal murine endogenous Aβ40 and Aβ42 levels in APP sw/0 ; Pdgfrβ +/− mice normally absent in APP sw/0 mice ( Fig. 3a,b ). At 9 months of age, murine Aβ contributed to 13 and 30% of total Aβ40 and Aβ42 levels found in brains of APP sw/0 ; Pdgfrβ +/− mice, respectively, compared with <1% in APP sw/0 ; Pdgfrβ +/+ controls ( Fig. 3c,d ), and co-localized with human Aβ in brain lesions ( Fig. 3e ). Pathological recruitment of endogenous Aβ has not been shown before in transgenic models of AD. Whether endogenous Aβ has a role in the progression of cerebral β-amyloidosis as reported previously for human Aβ [22] , [23] and/or endogenous prion protein in prion disease [24] remains to be determined. Nevertheless, these data indicate that pericytes have important functions in regulating human as well as murine Aβ metabolism. 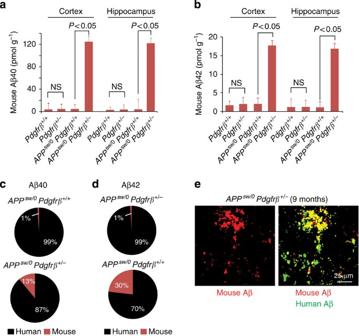Figure 3: Pericyte deficiency leads to the accumulation of murine Aβ inAPPsw/0Pdgfrβ+/−mice. (a–d) Murine Aβ40 and Aβ42 levels in the cortex and hippocampus (a,b) and contributions of human and murine Aβ40 and Aβ42 to total Aβ levels (c,d) in 9-month-oldAPPsw/0;Pdgfrβ+/+andAPPsw/0;Pdgfrβ+/−littermates. Ina,b, murine Aβ40 and Aβ42 levels were determined in 9-month-oldPdgfrβ+/+andPdgfrβ+/−mice. All values are means±s.e.m.,n=6 mice per group.P<0.05 by ANOVA followed by Tukey’spost-hoctests. Values inc,dderived from values given inFig. 3panelsa,bandFig. 1panelsa,b, based onn=6 mice per group. (e) Confocal microscopy analysis for the colocalization of murine endogenous Aβ (red) and human Aβ (green) in Aβ deposits in the cortex of 9-month-oldAPPsw/0;Pdgfrβ+/−mice. Images are representative findings from six mice per group. Scale bar, 25 μm. Figure 3: Pericyte deficiency leads to the accumulation of murine Aβ in APP sw/0 Pdgfrβ +/− mice. ( a – d ) Murine Aβ40 and Aβ42 levels in the cortex and hippocampus ( a , b ) and contributions of human and murine Aβ40 and Aβ42 to total Aβ levels ( c , d ) in 9-month-old APP sw/0 ; Pdgfrβ +/+ and APP sw/0 ; Pdgfrβ +/− littermates. In a , b , murine Aβ40 and Aβ42 levels were determined in 9-month-old Pdgfrβ +/+ and Pdgfrβ +/− mice. All values are means±s.e.m., n =6 mice per group. P <0.05 by ANOVA followed by Tukey’s post-hoc tests. Values in c , d derived from values given in Fig. 3 panels a , b and Fig. 1 panels a , b , based on n =6 mice per group. ( e ) Confocal microscopy analysis for the colocalization of murine endogenous Aβ (red) and human Aβ (green) in Aβ deposits in the cortex of 9-month-old APP sw/0 ; Pdgfrβ +/− mice. Images are representative findings from six mice per group. Scale bar, 25 μm. Full size image To determine whether loss of the Pdgfrβ allele can affect Aβ accumulation without the interaction with the APP sw/0 gene, we analysed Aβ levels in 9-month-old Pdgfrβ +/− and Pdgfrβ +/+ mice. In both Pdgfrβ +/− and Pdgfrβ +/+ mice, human Aβ was undetectable as expected ( Fig. 2a,b ) but murine brain Aβ40 and Aβ42 levels were comparable ( Fig. 3a,b ), suggesting that pericyte-deficient mice do not show a detectable accumulation of Aβ in the absence of the APP gene at an age when age-matched APP sw/0 ; Pdgfrβ +/− mice develop significant increases in both human and endogenous murine Aβ levels compared with their littermate APP sw/0 ; Pdgfrβ +/+ controls ( Figs 2a,b and 3a,b ). Lack of Aβ elevation in 9-month-old Pdgfrβ +/− mice may suggest that under physiological conditions of Aβ production low murine Aβ levels do not pose a significant challenge for Aβ clearance by pericytes, even when the pericyte pool was reduced by 26% ( Fig. 1b ). However, in 9-month-old human Aβ-overproducing APP sw/0 ; Pdgfrβ +/− mice, the 2–3 orders of magnitude-higher brain Aβ levels likely go above the clearance capability of the considerably diminished pericyte pool (that is, by 55%, Fig. 1b ), resulting in substantial human and murine Aβ accumulations. Pericytes control Aβ clearance in APP mice To determine whether pericyte deficiency affects Aβ clearance, brain interstitial fluid (ISF) Aβ levels were monitored by hippocampal in vivo microdialysis [25] , [26] in 3–4-month-old pericyte-deficient APP sw/0 ; Pdgfrβ +/− mice with a 31% loss of pericytes in the hippocampus; age-matched APP sw/0 ; Pdgfrβ +/+ controls have no loss of pericytes at this time point ( Fig. 1b ). Our data indicate a significant 2.4- and 2.7-fold increase in the steady-state levels of soluble Aβ40 and Aβ42 in brain ISF of APP sw/0 ; Pdgfrβ +/− mice compared with age-matched APP sw/0 ; Pdgfrβ +/+ littermates, respectively ( Fig. 4a,b ). The half-life of Aβ40 and Aβ42 in brain ISF [26] was increased in APP sw/0 ; Pdgfrβ +/− mice compared with APP sw/0 ; Pdgfrβ +/+ controls from 1.3 to 2.2 h, and 1.5 to 2.4 h, respectively ( Fig. 4c ), suggesting that the increase in ISF Aβ levels was because of diminished Aβ clearance. Importantly, an increase in Aβ ISF levels preceded Aβ and amyloid deposition in APP sw/0 ; Pdgfrβ +/− mice that were absent at 3–4 months of age ( Fig. 4d,e ) but were begin to accumulate at 6 months of age ( Supplementary Fig. S1a,b ) and correlated with a more pronounced 39% loss of pericytes ( Fig. 1b ). In support of our findings that pericyte deficiency leads to diminished Aβ clearance, we show that Aβ production and processing [14] are not affected by pericyte degeneration in APP sw/0 ; Pdgfrβ +/− mice, as indicated by unchanged levels of APP, comparable β-secretase activity and unchanged levels of sAPPβ, a soluble form of APP cleaved by β-secretase ( Fig. 4f–h ). 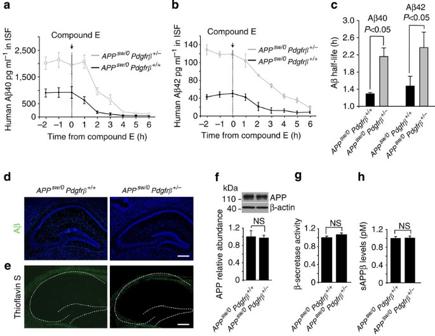Figure 4: ISF levels of Aβ increase in pericyte-deficientAPPsw/0Pdgfrβ+/−mice prior to Aβ deposition. (a,b) ISF Aβ40and Aβ42levels monitored byin vivohippocampal microdialysis of 3- to 4-month-oldAPPsw/0;Pdgfrβ+/−mice and age-matchedAPPsw/0;Pdgfrβ+/+littermates. Baseline Aβ levels were monitored for 3 h. (c) The elimination half-life of ISF Aβ was determined after administration of compound E (20 mg kg−1intraperitoneally). Values are means±s.e.m.,n=6 mice per group. In (c),P<0.05 by ANOVA followed by Tukey’spost-hoctests. (d,e) Representative cortex and hippocampus sections stained for Aβ (d) and thioflavin-S (e) in 3- to 4-month-oldAPPsw/0;Pdgfrβ+/+andAPPsw/0;Pdgfrβ+/−mice. Scale bar, 100 μm. (f–h) APP abundance relative to β-actin (f), β-secretase activity (g) and sAPPβ levels (h) in forebrain tissue from 6-month-oldAPPsw/0;Pdgfrβ+/−and age-matchedAPPsw/0;Pdgfrβ+/+littermates. Inf, values are means±s.e.m.,n=4 mice per group. Full-size blots are available in theSupplementary Fig. S5. Ing,h, values are means±s.e.m.,n=6 mice per group. NS, nonsignificant by Student’st-test. Figure 4: ISF levels of Aβ increase in pericyte-deficient APP sw/0 Pdgfrβ +/− mice prior to Aβ deposition. ( a , b ) ISF Aβ 40 and Aβ 42 levels monitored by in vivo hippocampal microdialysis of 3- to 4-month-old APP sw/0 ; Pdgfrβ +/− mice and age-matched APP sw/0 ; Pdgfrβ +/+ littermates. Baseline Aβ levels were monitored for 3 h. ( c ) The elimination half-life of ISF Aβ was determined after administration of compound E (20 mg kg −1 intraperitoneally). Values are means±s.e.m., n =6 mice per group. In ( c ), P <0.05 by ANOVA followed by Tukey’s post-hoc tests. ( d , e ) Representative cortex and hippocampus sections stained for Aβ ( d ) and thioflavin-S ( e ) in 3- to 4-month-old APP sw/0 ; Pdgfrβ +/+ and APP sw/0 ; Pdgfrβ +/− mice. Scale bar, 100 μm. ( f – h ) APP abundance relative to β-actin ( f ), β-secretase activity ( g ) and sAPPβ levels ( h ) in forebrain tissue from 6-month-old APP sw/0 ; Pdgfrβ +/− and age-matched APP sw/0 ; Pdgfrβ +/+ littermates. In f , values are means±s.e.m., n =4 mice per group. Full-size blots are available in the Supplementary Fig. S5 . In g , h , values are means±s.e.m., n =6 mice per group. NS, nonsignificant by Student’s t -test. Full size image We next show that primary cultured murine brain pericytes [6] rapidly clear extracellular Cy3-labelled Aβ40 via low-density lipoprotein receptor-related protein 1 (LRP1), a key Aβ clearance receptor in brain vasculature [8] , [21] , [27] , that is normally expressed in brain pericytes in vivo ( Fig. 5a ). LRP1-mediated Aβ clearance by cultured pericytes has been demonstrated by administering antibodies to block the function of specific LDL receptors ( Fig. 5b,c ) and by quantifying the effects of silencing different LDL receptors with specific siRNA-blocking agents [6] ( Fig. 5d,e ). Moreover, adenoviral-mediated re-expression of human LRP1 minigene rescued the ability of pericytes with siRNA-induced LRP1 knockdown to clear Aβ ( Fig. 5e ). Excessive LRP1-mediated accumulation of Aβ in pericytes over longer periods of time such as 7 days resulted in cell death ( Fig. 5f ) similar to as reported in human brain pericyte cultures [28] . These findings not only suggest that Aβ clearance by pericytes is critical for Aβ homeostasis but also show that extreme Aβ accumulation in pericytes leads to cell death. We next show in vivo that Aβ-overproducing APP sw/0 mice have an age-dependent loss of pericytes from 17% at 9 months of age ( Fig. 1b ) to 35% at 18 months of age as reported by another study [29] . Thus, with age Aβ progressively depletes the pericyte pool, thereby increasing the Aβ load on the remaining pericytes, possibly establishing a propagating negative spiral that accelerates disease progression. 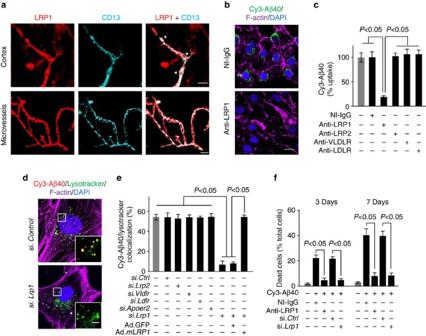Figure 5: Rapid clearance of Cy3-Aβ40 by murine brain pericytes and cell death after prolonged Aβ accumulation. (a) Colocalization of low-density LRP1 (red) and pericyte marker CD13 (Cyan) in brain microvessels in the mouse cortex tissue section (upper panels) and in freshly isolated microvessels from the mouse brain (bottom panels). *, pericyte cell bodies. Scale bar, 20 μm. (b,c) Cy3-Aβ40 uptake by cultured murine brain pericytes determined within 30 min in the presence of non-immune IgG (NI-IgG) and LRP1-specific blocking antibody (b, scale bar, 10 μm) and quantification of Cy3-Aβ40 pericyte uptake with and without NI-IgG, LRP1-, low-density LRP2-, very low-density lipoprotein receptor (VLDLR)- and low-density lipoprotein receptor (LDLR)-specific antibodies (c). Uptake in the absence of antibodies was arbitrarily taken as 100%. Mean±s.e.m.,n=3 independent cultures per group. (d,e) Cy3-Aβ40 internalization and lysosomal colocalization in pericytes 48 h after siRNA silencing ofLrp1or control siRNA (siCtrl) (d, scale bar, 10 μm) and quantification of Cy3-Aβ40 and lysotraker colocalization in pericytes after silencing ofLrp2,Vldlr,Ldlr,Apoer2andLrp1and adenoviral-mediated re-expression of theLRP1minigene (Ad.mLRP1) (e). GFP, green fluorescent protein. Mean±s.e.m.,n=3 independent cultures per group. (f) Pericyte cell death after 3 and 7 days of Aβ40 accumulation. Cells were cultured with and without 5 μM Aβ40 for 3 and 7 days in the presence and absence of NI-IgG and anti-LRP1 and after siLrp1silencing or siCtrl.Mean±s.e.m.,n=3 independent cultures per group. Inc,e,f, all comparisons are by ANOVA followed by Tukey’spost-hoctests. Figure 5: Rapid clearance of Cy3-Aβ40 by murine brain pericytes and cell death after prolonged Aβ accumulation. ( a ) Colocalization of low-density LRP1 (red) and pericyte marker CD13 (Cyan) in brain microvessels in the mouse cortex tissue section (upper panels) and in freshly isolated microvessels from the mouse brain (bottom panels). *, pericyte cell bodies. Scale bar, 20 μm. ( b , c ) Cy3-Aβ40 uptake by cultured murine brain pericytes determined within 30 min in the presence of non-immune IgG (NI-IgG) and LRP1-specific blocking antibody ( b , scale bar, 10 μm) and quantification of Cy3-Aβ40 pericyte uptake with and without NI-IgG, LRP1-, low-density LRP2-, very low-density lipoprotein receptor (VLDLR)- and low-density lipoprotein receptor (LDLR)-specific antibodies ( c ). Uptake in the absence of antibodies was arbitrarily taken as 100%. Mean±s.e.m., n =3 independent cultures per group. ( d , e ) Cy3-Aβ40 internalization and lysosomal colocalization in pericytes 48 h after siRNA silencing of Lrp1 or control siRNA (si Ctrl ) ( d , scale bar, 10 μm) and quantification of Cy3-Aβ40 and lysotraker colocalization in pericytes after silencing of Lrp2 , Vldlr , Ldlr , Apoer2 and Lrp1 and adenoviral-mediated re-expression of the LRP1 minigene (Ad.m LRP1 ) ( e ). GFP, green fluorescent protein. Mean±s.e.m., n =3 independent cultures per group. ( f ) Pericyte cell death after 3 and 7 days of Aβ40 accumulation. Cells were cultured with and without 5 μM Aβ40 for 3 and 7 days in the presence and absence of NI-IgG and anti-LRP1 and after si Lrp1 silencing or si Ctrl. Mean±s.e.m., n =3 independent cultures per group. In c , e , f , all comparisons are by ANOVA followed by Tukey’s post-hoc tests. Full size image The relative levels of LRP1 expression in brain microvessels and pericytes isolated from APP sw/0 ; Pdgfrβ +/− mice and APP sw/0 ; Pdgfrβ +/+ littermate controls were comparable ( Supplementary Fig. S2a,b ), suggesting that LRP1 cellular expression is not altered by partial Pdgfrβ gene deletion in pericytes. However, the number of pericytes was significantly reduced by 31% in 9-month-old APP sw/0 ; Pdgfrβ +/− mice compared with age-matched APP sw/0 ; Pdgfrβ +/+ littermate controls ( Fig. 1b ). Collectively, these data suggest that total amount of LRP in the pericyte pool that is available for clearance of Aβ in APP sw/0 ; Pdgfrβ +/− mice is significantly diminished compared with APP sw/0 ; Pdgfrβ +/+ mice because of the reduced number of pericytes rather than diminished LRP1 cellular expression in Pdgfrβ -deficient pericytes. APP sw/0 ; Pdgfrβ +/− mice did not show changes in brain microvascular expression of other known Aβ transporters such as P-glycoprotein and receptor for advanced age glycation products [2] ( Supplementary Fig. S2c,d ) or changes in the levels of Aβ-degrading enzymes in the brain—that is, insulin-degrading enzyme and neprilysin—compared with APP sw/0 ; Pdgfrβ +/+ controls ( Supplementary Fig. S2e,f ), thus ruling out these mechanisms as contributory to increased Aβ levels observed in pericyte-deficient APP sw/0 ; Pdgfrβ +/− mice. The levels of PDGFRβ receptor in brain microvessels of APP sw/0 ; Pdgfrβ +/+ and age-matched Pdgfrβ +/+ littermate controls were comparable, suggesting that accumulation of Aβ does not influence the expression of PDGFRβ ( Supplementary Fig. S2g,h ). On the other hand, there was ~65% reduction in PDGFRβ in brain microvessels of APP sw/0 ; Pdgfrβ +/− mice compared with APP sw/0 ; Pdgfrβ +/+ controls ( Supplementary Fig. S2g,h ) indicating that after crossing with Pdgfrβ +/− mice APP sw/0 mice develop a severe PDGFRβ deficiency, which contributes to accelerated pericyte loss compared with more moderate losses in Pdgfrβ +/− mice alone or APP sw/0 mice alone ( Fig. 1b ). APP sw/0 mice develop high plasma Aβ levels, raising a possibility that plasma Aβ may contribute and increase brain Aβ levels by their transport across the blood–brain barrier [30] . The exact contributions of plasma-derived and brain-derived Aβ to total brain Aβ in APP sw/0 mice remain, however, unknown. Our data in APP sw/0 ; Pdgfrβ +/− mice compared with APP sw/0 ; Pdgfrβ +/+ littermate controls show a significant increase in the half-life of soluble Aβ in brain ISF after inhibition of Aβ production, suggesting that reduced Aβ clearance [26] , [27] mediates Aβ accumulation in pericyte-deficient APP mice. To validate our findings in an APP model with low plasma Aβ levels, we have performed a limited number of experiments in Pdgfrβ +/− mice crossed with transgenic Dutch/Iowa mice ( APP swDI ) expressing low levels of human APP under control of Thy 1.2 neuronal promoter harbouring Swedish mutation and the Dutch and Iowa vasculotropic Aβ mutations [27] , [31] . APP swDI mice express human APP exclusively in neurons and have extremely low plasma Aβ levels (<30 pM) [31] , thereby ruling out a possibility of any significant contribution of plasma Aβ transport to the elevated brain Aβ levels. Notably, APP swDI mice exhibit earlier onset and more robust Aβ pathology than APP sw/0 mice because the Dutch/Iowa Aβ mutant peptides produced by these mice are poorly cleared from the brain and at the blood–brain barrier compared with their respective wild-type Aβ40 and Aβ42 isoforms produced by APP sw/0 mice, as we reported [27] . After 5 months, pericyte-deficient APP swDI ; Pdgfrβ +/− mice had approximately seven- to eightfold greater Aβ load in the cortex and hippocampus compared with APP swDI ; Pdgfrβ +/+ littermate controls ( Fig. 6a,b ). These data suggest that pericyte loss worsens Aβ clearance in APP mice regardless of whether plasma Aβ levels are high as in APP sw/0 mice [30] or extremely low as in APP swDI mice [27] , [31] , and that the effect of pericytes on Aβ clearance from the brain rather than on plasma Aβ has a major role in accelerating Aβ pathology in APP mice. 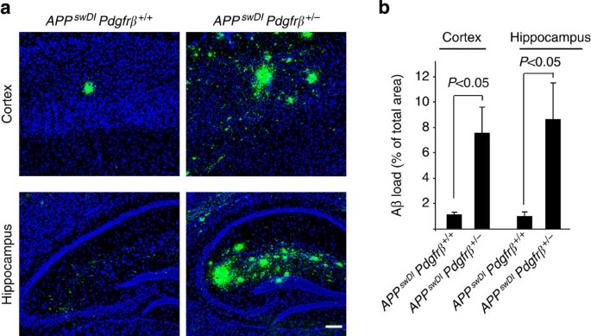Figure 6: Accelerated Aβ pathology inAPPswDIPdgfrβ+/−mice. (a) Representative cortex and hippocampus sections stained with antibody against Aβ (6E10; green) and nuclei (blue) in 5-month-oldAPPswDI;Pdgfrβ+/+andAPPswDI;Pdgfrβ+/−mouse. Scale bar, 100 μm. (b) Quantification of Aβ load in the cortex and hippocampus of 5-month-oldAPPswDI;Pdgfrβ+/+andAPPswDI;Pdgfrβ+/−mice. Mean+s.e.m.,n=5 mice per group.P<0.05 by Student’st-test. Figure 6: Accelerated Aβ pathology in APP swDI Pdgfrβ +/− mice. ( a ) Representative cortex and hippocampus sections stained with antibody against Aβ (6E10; green) and nuclei (blue) in 5-month-old APP swDI ; Pdgfrβ +/+ and APP swDI ; Pdgfrβ +/− mouse. Scale bar, 100 μm. ( b ) Quantification of Aβ load in the cortex and hippocampus of 5-month-old APP swDI ; Pdgfrβ +/+ and APP swDI ; Pdgfrβ +/− mice. Mean+s.e.m., n =5 mice per group. P <0.05 by Student’s t -test. Full size image Pericyte loss triggers tau pathology in APP sw/0 mice Next, we studied whether pericyte loss can influence the development of tau pathology and neurodegenerative changes in APP sw/0 mice. Our immunocytochemical analysis in APP sw/0 ; Pdgfrβ +/− mice shows that pericyte loss leads to a significant tau hyperphosphorylation in cortical and hippocampal neurons ( Fig. 7a–d ), appearance of caspase-cleaved tau in neurons that has been shown to facilitate nucleation-dependent tau filament formation [32] and conformational changes in tau as shown with the early pathological tau marker MC1 [32] ( Fig. 7e,f ) also confirmed using ELISA for insoluble tau (not shown). Notably, changes in tau pathology were not observed in age-matched control APP sw/0 ; Pdgfrβ +/+ mice ( Fig. 7a–e ) or Pdgfrβ +/− mice ( Supplementary Fig. S3a,b ) and/or older APP sw/0 ; Pdgfrβ +/+ mice ( Supplementary Fig. S3c,d ) with brain Aβ40 and Aβ42 levels comparable to those found in younger 9-month-old pericyte-deficient APP sw/0 ; Pdgfrβ +/− mice. These data suggest that Aβ alone and/or moderate pericyte deficiency alone causing vascular damage and blood–brain barrier breakdown [5] are not sufficient to trigger early tau pathology, which we show requires a combined action of the two hits as illustrated in APP sw/0 ; Pdgfrβ +/− mice. 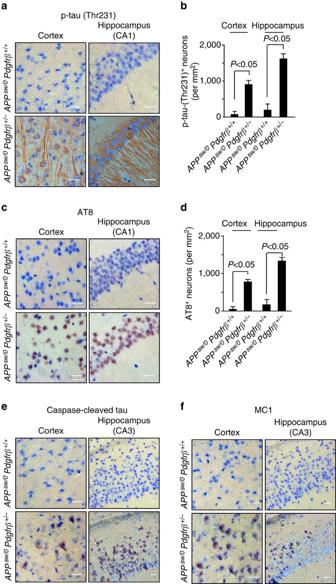Figure 7: Tau pathology in pericyte-deficientAPPsw/0Pdgfrβ+/−mice. (a–f) Representative cortex and hippocampus sections stained with antibodies against p-tau (Thr231) (a), quantification of p-tau (Thr231)-positive neurons (b), p-tau (Ser202/Thr205, AT8) (c), quantification of AT8-positive neurons (d), caspase-cleaved tau (e) and an early pathological tau marker MC1 (f) in 9-month-oldAPPsw/0Pdgfrβ+/−mice and age-matchedAPPsw/0Pdgfrβ+/+littermates. Ina,c,e,f, scale bar, 25 μm. CA1 and CA3 denote hippocampal regions. Inb,d, values are means±s.e.m.,n=5 mice per group.P<0.05 by ANOVA followed by Tukey’spost-hoctests. Figure 7: Tau pathology in pericyte-deficient APP sw/0 Pdgfrβ +/− mice. ( a – f ) Representative cortex and hippocampus sections stained with antibodies against p-tau (Thr231) ( a ), quantification of p-tau (Thr231)-positive neurons ( b ), p-tau (Ser202/Thr205, AT8) ( c ), quantification of AT8-positive neurons ( d ), caspase-cleaved tau ( e ) and an early pathological tau marker MC1 ( f ) in 9-month-old APP sw/0 Pdgfrβ +/− mice and age-matched APP sw/0 Pdgfrβ +/+ littermates. In a , c , e , f , scale bar, 25 μm. CA1 and CA3 denote hippocampal regions. In b , d , values are means±s.e.m., n =5 mice per group. P <0.05 by ANOVA followed by Tukey’s post-hoc tests. Full size image Pericyte loss leads to early neuronal loss in APP sw/0 mice Importantly, pericyte deficiency led to progressive neuronal degenerative changes as evidenced by ~50% reductions in the neurite density and 23–25% loss of neurons in the cortex and hippocampus in 9-month-old APP sw/0 ; Pdgfrβ +/− mice compared with their respective age-matched APP sw/0 ; Pdgfrβ +/+ littermate controls ( Fig. 8a–c ). In the absence of the APP transgene, pericyte deficiency leads, however, to only modest 8% loss of neurons in Pdgfrβ +/− mice as reported previously [5] , whereas APP sw/0 mice did not show neuronal loss at the same age ( Fig. 8a,c ). Consistent with significant neurodegenerative changes, 9-month-old pericyte-deficient APP sw/0 ; Pdgfrβ +/− mice performed poorly on several hippocampal-dependent behavioural tests including burrowing, nest construction and novel object location compared with their age-matched APP sw/0 ; Pdgfrβ +/+ littermate controls or Pdgfrβ +/− mice of the corresponding age ( Fig. 8d–f ). 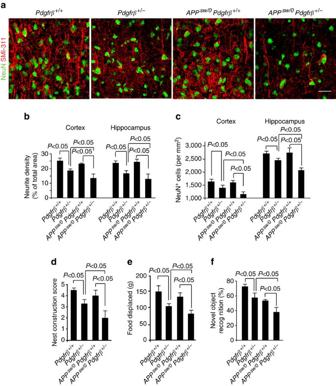Figure 8: Neuronal degeneration inAPPsw/0Pdgfrβ+/−mice. (a,b) Representative confocal microscopy analysis of SMI311-positive neurofilaments and NeuN-positive hippocampal neurons (a) and quantification of SMI311-positive neurofilaments (b) and NeuN-positive neurons (c) in the cortex and hippocampus of 9-month-old age-matchedPdgfrβ+/+, Pdgfrβ+/−,APPsw/0;Pdgfrβ+/+andAPPsw/0;Pdgfrβ+/−littermates mice. Ina, scale bar, 25 μm. Inb,c, values are means±s.e.m.,n=6 mice per group.P<0.05 by ANOVA followed by Tukey’spost-hoctests. (d–f) Behavioural analysis of nest construction (d), burrowing (e) and novel object location (f) in 9-month-oldPdgfrβ+/+, Pdgfrβ+/−,APPsw/0;Pdgfrβ+/+andAPPsw/0;Pdgfrβ+/−age-matched littermate mice. Ind–f, values are means±s.e.m.,n=6 mice per group.P<0.05 by ANOVA followed by Tukey’spost-hoctests. Figure 8: Neuronal degeneration in APP sw/0 Pdgfrβ +/− mice. ( a , b ) Representative confocal microscopy analysis of SMI311-positive neurofilaments and NeuN-positive hippocampal neurons ( a ) and quantification of SMI311-positive neurofilaments ( b ) and NeuN-positive neurons ( c ) in the cortex and hippocampus of 9-month-old age-matched Pdgfrβ +/+ , Pdgfrβ +/− , APP sw/0 ; Pdgfrβ +/+ and APP sw/0 ; Pdgfrβ +/− littermates mice. In a , scale bar, 25 μm. In b , c , values are means±s.e.m., n =6 mice per group. P <0.05 by ANOVA followed by Tukey’s post-hoc tests. ( d – f ) Behavioural analysis of nest construction ( d ), burrowing ( e ) and novel object location ( f ) in 9-month-old Pdgfrβ +/+ , Pdgfrβ +/− , APP sw/0 ; Pdgfrβ +/+ and APP sw/0 ; Pdgfrβ +/− age-matched littermate mice. In d – f , values are means±s.e.m., n =6 mice per group. P <0.05 by ANOVA followed by Tukey’s post-hoc tests. Full size image At an early 1 month of age, a modest 17% pericyte loss in APP sw/0 ; Pdgfrβ +/− mice compared with no loss in APP sw/0 ; Pdgfrβ +/+ controls (Fig. 1b) did not affect Aβ levels, tau hyperphoshorylation, neurite density and/or number of neurons (Supplementary Fig. S4a–f). Measurements of sensorimotor cortex activity in response to hindlimb stimulation determined by in vivo voltage-sensitive dye (VSD) imaging in 1- to 2-month-old APP sw/0 ; Pdgfrβ +/− mice ( Supplementary Fig. S4g–i ) indicated no changes in cortical activity as shown by comparable time-lapse imaging profiles of the spreading of depolarization and no changes in the peak of VSD amplitude and/or time-to-peak of the depolarization wave. Consistent with these findings, no behavioural changes were noticed in 1- to 2-month-old APP sw/0 ; Pdgfrβ +/− mice ( Supplementary Fig. S4j,k ). Vascular damage in pericyte-deficient APP sw/0 mice An early and progressive blood–brain barrier breakdown and microvascular reductions have been described in pericyte-deficient mice [3] , [4] , [5] and APP sw/0 mice [8] , [33] as well as in AD individuals [8] , [10] , [11] , [12] , [13] and have also been shown at an early stage in 1-month-old pericyte-deficient APP sw/0 ; Pdgfrβ +/− mice compared with APP sw/0 ; Pdgfrβ +/+ control mice, as indicated by a eightfold increase in vascular leakage of immunoglobulin G ( Fig. 9a,b ) and 29% decrease in the total capillary length ( Fig. 9c ). At this early stage, APP sw/0 ; Pdgfrβ +/− mice also developed a twofold greater accumulation of immunoglobulin G (IgG) and 12% greater microvascular reductions compared with Pdgfrβ +/− mice, respectively ( Fig. 9b,c ). This initial vascular damage did not affect, however, neuronal function ( Supplementary Fig. S4 ) that is consistent with previous reports [5] , [6] . At a later stage, the degree of blood–brain barrier breakdown as indicated by the magnitude of IgG extravascular deposition and reductions in the capillary length became more pronounced and remained significantly greater in APP sw/0 ; Pdgfrβ +/− mice compared to either APP sw/0 ; Pdgfrβ +/+ mice or Pdgfrβ +/− mice alone ( Fig. 9d–f ). Significant microvascular reductions in APP sw/0 ; Pdgfrβ +/− mice can reduce the surface area for transvascular and perivascular Aβ clearance, which may additionally contribute to reduced Aβ elimination from the brain. Our findings are consistent with a concept that pericyte degeneration causing accelerated vascular damage from one end, and accelerated Aβ accumulation from the other, creates a double hit in brains of pericyte-deficient APP sw/0 ; Pdgfrβ +/− mice that leads to severe tau pathology ( Fig. 7a–f ), neuronal loss ( Fig. 8a,c ) and cognitive changes ( Fig. 8d–f ). 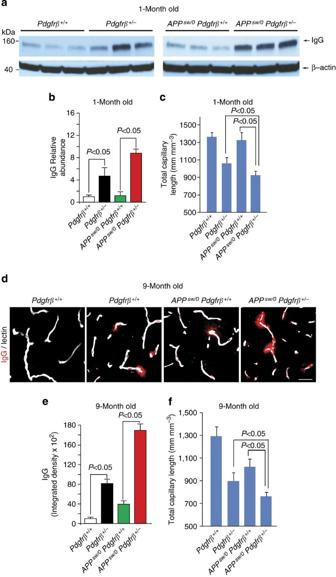Figure 9: Accelerated blood–brain barrier breakdown and microvascular reductions in pericyte-deficientAPPsw/0Pdgfrβ+/−mice. (a,b) Western blot analysis of serum IgG in capillary-depleted cortical homogenates relative to β-actin (a) and quantification of IgG extravascular levels (b) in 1-month-oldPdgfrβ+/+, Pdgfrβ+/−,APPsw/0;Pdgfrβ+/+andAPPsw/0;Pdgfrβ+/−mice. Full-size blots can be found inSupplementary Fig. S5. (c) Total length of lectin-positive capillary profiles in 1-month-oldPdgfrβ+/+, Pdgfrβ+/−,APPsw/0;Pdgfrβ+/+andAPPsw/0;Pdgfrβ+/−mice. Inb, values are means±s.e.m.,n=4 mice per group. Inc, values are means±s.e.m.,n=6 mice per group.P<0.05 by ANOVA followed by Tukey’spost-hoctests. (d,e) IgG extravascular leakage (d, scale bar, 100 μm) and quantification of IgG extravascular deposits (e) in 9-month-oldPdgfrβ+/+, Pdgfrβ+/−,APPsw/0;Pdgfrβ+/+andAPPsw/0;Pdgfrβ+/−mice.(f) Total length of lectin-positive capillary profiles in 9-month-oldPdgfrβ+/+, Pdgfrβ+/−,APPsw/0;Pdgfrβ+/+andAPPsw/0;Pdgfrβ+/−mice. Ine,f, values are means±s.e.m.,n=6 mice per group.P<0.05 by ANOVA followed by Tukey’spost-hoctests. Figure 9: Accelerated blood–brain barrier breakdown and microvascular reductions in pericyte-deficient APP sw/0 Pdgfrβ +/− mice. ( a , b ) Western blot analysis of serum IgG in capillary-depleted cortical homogenates relative to β-actin ( a ) and quantification of IgG extravascular levels ( b ) in 1-month-old Pdgfrβ +/+ , Pdgfrβ +/− , APP sw/0 ; Pdgfrβ +/+ and APP sw/0 ; Pdgfrβ +/− mice. Full-size blots can be found in Supplementary Fig. S5 . ( c ) Total length of lectin-positive capillary profiles in 1-month-old Pdgfrβ +/+ , Pdgfrβ +/− , APP sw/0 ; Pdgfrβ +/+ and APP sw/0 ; Pdgfrβ +/− mice. In b , values are means±s.e.m., n =4 mice per group. In c , values are means±s.e.m., n =6 mice per group. P <0.05 by ANOVA followed by Tukey’s post-hoc tests. ( d , e ) IgG extravascular leakage ( d , scale bar, 100 μm) and quantification of IgG extravascular deposits ( e ) in 9-month-old Pdgfrβ +/+ , Pdgfrβ +/− , APP sw/0 ; Pdgfrβ +/+ and APP sw/0 ; Pdgfrβ +/− mice. ( f ) Total length of lectin-positive capillary profiles in 9-month-old Pdgfrβ +/+ , Pdgfrβ +/− , APP sw/0 ; Pdgfrβ +/+ and APP sw/0 ; Pdgfrβ +/− mice. In e , f , values are means±s.e.m., n =6 mice per group. P <0.05 by ANOVA followed by Tukey’s post-hoc tests. Full size image Collectively, our findings suggest that accelerated pericyte loss in APP sw/0 mice because of aberrant PDGFRβ signalling in pericytes influences several steps within the AD pathogenic cascade by generating multiple negative downstream spiral effects, as illustrated in Fig. 10 . From one end, pericyte loss diminishes early in the disease process clearance of soluble Aβ accelerating accumulation and deposition of Aβ in the brain, which in turn self-amplifies Aβ-induced pericyte loss in a negative spiral. From the other end, loss of pericytes disrupts cerebrovascular integrity and leads to microvascular reductions amplifying vascular damage. Together, these two hits act in parallel to lead to the development of a complete spectrum of AD pathology including, in addition to accelerated Aβ accumulation, the appearance of tau pathology, neuronal degeneration and loss. 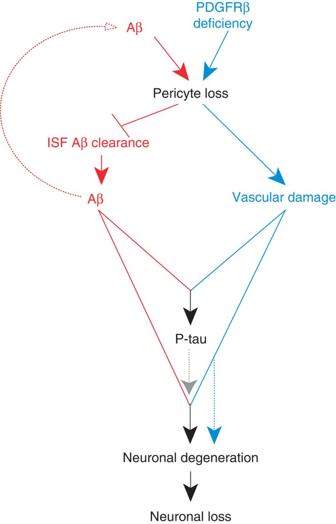Figure 10: Pericyte loss influences multiple steps of Alzheimer’s-like pathogenic cascade inAPPsw/0mice. Within the Aβ pathway (red), pericyte loss inAPPsw/0mice because of PDGFRβ deficiency and/or excessive accumulation of Aβ in pericytes diminishes early in the disease process clearance of soluble Aβ from brain ISF causing an early Aβ accumulation and deposition in the brain, which in turn amplifies the loss of pericytes. Within the vasculature, an Aβ-independent pathway driven by aberrant PDGFRβ signalling in pericytes (blue) leads to accelerated pericyte loss that amplifies blood–brain barrier disruption and microvascular reductions inAPPsw/0mice and the degree of vascular damage. Both pathways acting in parallel lead to an early development of a full spectrum of AD-like pathology in mice including significant Aβ pathology, tau pathology, neuronal degeneration and neuronal loss that are not observed either within the Aβ pathway alone or the vascular Aβ-independent pathway alone. Figure 10: Pericyte loss influences multiple steps of Alzheimer’s-like pathogenic cascade in APP sw/0 mice. Within the Aβ pathway (red), pericyte loss in APP sw/0 mice because of PDGFRβ deficiency and/or excessive accumulation of Aβ in pericytes diminishes early in the disease process clearance of soluble Aβ from brain ISF causing an early Aβ accumulation and deposition in the brain, which in turn amplifies the loss of pericytes. Within the vasculature, an Aβ-independent pathway driven by aberrant PDGFRβ signalling in pericytes (blue) leads to accelerated pericyte loss that amplifies blood–brain barrier disruption and microvascular reductions in APP sw/0 mice and the degree of vascular damage. Both pathways acting in parallel lead to an early development of a full spectrum of AD-like pathology in mice including significant Aβ pathology, tau pathology, neuronal degeneration and neuronal loss that are not observed either within the Aβ pathway alone or the vascular Aβ-independent pathway alone. Full size image Our data suggest that neither Aβ on its own nor a partial Pdgfrβ genetic deletion alone causing a moderate loss of pericytes [4] , [5] , [7] can trigger tau pathology and a substantive neuronal loss as seen at an early disease stage in double transgenic APP sw/0 ; Pdgfrβ +/− mice. We and others have previously reported that Pdgfrβ +/− mice do not express detectable levels of PDGFRβ in neurons and/or other cell types of the neurovascular unit including astrocytes and endothelial cells [4] , [5] , [34] , [35] . In addition, it is well established that loss of PDGF-BB/PDGFRβ signalling because of partial and/or global Pdgfb and/or Pdgfrβ gene deletion or malfunction results in vascular phenotype in the central nervous system caused by loss of pericytes, not neuronal loss [3] , [4] , [5] , [35] , [36] . These data suggest that increased Aβ burden, tau pathology and neuronal loss that are observed in double transgenic APP sw/0 ; Pdgfrβ +/− mice cannot be attributed to a downstream effect of PDGFRβ signalling in neurons and/or astrocytes that is independent of vascular pericytes. The present data support the two-hit vascular hypothesis of AD [8] , suggesting that vascular damage (in the present study a deficiency in vascular pericytes) and Aβ act in parallel to initiate and/or accelerate a chronic neurodegenerative disorder. Interestingly, intracellular accumulation of Aβ alone at the levels that exceed Aβ clearance capability of pericytes leads to pericyte cell death both in vitro and in vivo , which might be particularly relevant to degeneration and loss of pericytes in sporadic AD [8] , [11] , [12] , [13] . In summary, we show that brain pericytes control an AD-like neurodegenerative process in APP sw/0 mice and therefore may represent a novel therapeutic target to modify disease progression in AD. Future studies should explore whether pericyte rescue by re-expression of the Pdgfrβ gene will slow down Alzheimer-like neurodegeneration cascade in APP sw/0 ; Pdgfrβ +/− mice with accelerated pericyte loss. Although our data show that accumulation of Aβ in APP sw/0 ; Pdgfrβ +/+ mice does not reduce PDGFRβ levels in brain microvessels compared with control Pdgfrβ +/+ mice, future studies should determine whether Aβ accumulation in pericytes in APP sw/0 mice and AD individuals can lead to functional changes in PDGF-BB signal transduction to PDGFRβ in pericytes that might trigger pericyte loss without affecting PDGFRβ levels. Search for molecular cues that cause loss of pericytes in AD models and AD may ultimately lead to the discovery of new therapeutics to control pericyte loss and consequently slow down the pathogenic neurodegeneration cascade in AD. Animals Mice were housed in plastic cages on a 12-h light cycle with ad libitum access to water and a standard laboratory diet. All procedures were approved by the Institutional Animal Care and Use Committee at the University of Southern California and the University of Rochester with National Institutes of Health guidelines. Pdgfrβ +/− was generated as previously described [5] , [37] . APP sw/0 mice expressing human APP transgene with the K670M/N671L (Swedish) double mutation under control of the hamster prion promoter [19] were crossed with Pdgfrβ +/− mice to generate pericyte-deficient APP sw/0 ; Pdgfrβ +/− mice and their corresponding littermate controls. In a limited number of experiments, Pdgfrβ +/− mice were crossed with transgenic Dutch/Iowa mice ( APP swDI ) expressing low levels of human APP under control of Thy 1.2 neuronal promoter harbouring Swedish mutation and the Dutch and Iowa vasculotropic Aβ mutations [27] , [31] . To minimize confounding effects of background heterogeneity, all experiments were performed using age-matched littermates. All the animals were included in the study. In all experiments, we used animals of both sexes. Pdgfrβ +/+ , Pdgfrβ +/− , APP sw/0 ; Pdgfrβ +/+ and APP sw/0 ; Pdgfrβ +/− mice were 1, 3, 6 and 9 months old. APP swDI ; Pdgfrβ +/+ and APP swDI ; Pdgfrβ +/− mice were 5 months old. All animals were randomized for their genotype information. All experiments were blinded; the operators responsible for experimental procedure and data analysis were blinded and unaware of group allocation throughout the experiments. Multiphoton imaging One day before imaging animals received an intraperitoneal injection of 10 mg kg −1 methoxy-X04 (Neuroptix, Acton, MA, USA). The following day the mice were anesthetized using initially 5% isoflurane, and then within 15–30 s mice were placed on a heating pad (37 °C) and maintained under anesthesia using a face mask with a continuous delivery of air containing 1.3–1.5% isoflurane. The cranium was firmly secured in a stereotaxic frame. A high-speed dental drill (tip FST 19007-05, Fine Science Tools Inc., Foster City, CA, USA) was used to thin a square cranial window about 2 × 2 mm over the parietal cortex, and 45 degree forceps were used to remove the square piece of skull. Gelfoam (Pharmacia & Upjohn Company, Kalamazoo, MA, USA) was applied immediately to control any cranial or dural bleeding. A sterile 5-mm glass cover slip was then placed on the dura mater and sealed with a 1:1 mixture of bone cement and cyanoacrylate-based glue. Texas-Red-conjugated Dextran (70 kDa; 200 mg kg −1 ) was injected via tail vein in order to create a fluorescent angiogram. In vivo images were acquired using a Zeiss 5MP multiphoton microscope coupled to a 900-nm mode locked Ti:sapphire laser (Mai Tai, Spectra Physics, Santa Clara, CA, USA) [21] . Quantification of residual X04 fluorescence was analysed using the NIH Image J software. Confocal microscopy All images were taken with a Zeiss 510 confocal microscopy and analysed using the NIH Image J software [5] , [6] , [21] . Briefly, the number of CD13-positive pericytes and NeuN-positive neurons were analysed using the Image J cell counter tool and expressed per mm 2 of total tissue area. The length of capillaries ( ⩽ 6 μm in diameter) was measured using the Image J ‘Neuro J’ plug-in length analysis tool. The length of capillaries was expressed as mm of lectin-positive vascular profiles per mm 3 of brain tissue. To quantify extravascular IgG accumulations, the positive immunofluorescent IgG signals were subjected to threshold-processing and measured using the Image J-integrated density measurement tool. SMI-positive neurofilaments were subjected to threshold-processing and the area of positive neurites was calculated as a percentage of total tissue area. For the quantification of CD13-positive pericyte numbers, capillary length, IgG extravasation, neurite length and NeuN-positive cell numbers six randomly selected fields in the cortex (420 × 420 μm) and four randomly selected fields in the hippocampus (420 × 420 μm) per section from six non-adjacent (~100 μm apart) sections per animal were analysed. At least six animals per group were analysed. Quantification of Aβ load in the cortex and hippocampus was determined by the area occupied by Aβ-positive immunostaining using the NIH Image J software [21] , [38] . Tissue immunofluorescent and fluorescent thioflavin-S and lectin staining Mice were anesthetized as described above and transcardially perfused with phosphate buffered saline (PBS) containing 5 U ml −1 heparin. Brains were dissected and embedded into optimal cutting temperature compound (Tissue-Tek, Torrance, CA, USA) on dry ice. Optimal cutting temperature-embedded frozen brain tissue was cryosectioned at a thickness of 14–18 μm and subsequently fixed in ice-cold acetone. Sections were blocked with 5% normal swine serum (Vector Laboratories, Burlingame, CA, USA) for 60 min and incubated in primary antibody diluted in blocking solution overnight at 4 °C. We used the following primary antibodies: rabbit anti-human Aβ (Cell Signaling Technology; no. 8243; 1:200), mouse anti-mouse Aβ (Invitrogen; AMB0062; 1:200), goat anti-mouse PDGFRβ (R&D Systems; AF1042; 1:100), mouse anti-NeuN (Millipore; MAB377; 1:200), mouse anti-neurofilament SMI-311 (Abcam; ab24575; 1:1,000) and goat anti-CD13 (R&D Systems; AF2335; 1:200). Sections were washed in PBS and incubated with the following secondary antibodies: Alexa 488-conjugated donkey anti-rabbit (Invitrogen; A11008; 1:200) to detect human Aβ, Alexa 568-conjugated donkey anti-goat (Invitrogen; A11057; 1:200) to detect mouse neurofilament, PDGFRβ or CD13, Alexa 488-conjugated donkey anti-mouse (Invitrogen; A21202; 1:200) to detect NeuN. To visualize brain microvessels, sections were incubated with Dylight 488-conjugated L. esculentum lectin (Vector Laboratories; DL-1174; 1:100) and coverslipped with fluorescent mounting medium (Dako, Carpinteria, CA, USA). For thioflavin-S staining [21] , [38] , frozen brain sections (20 μm) were stained with 0.2% thioflavin-S in PBS for 10 min and washed three times with PBS before imaging. Bright field microscopy analysis Mice were transcardially perfused with 4% paraformaldehyde in 0.1 M PBS. Brains were postfixed in 4% paraformaldehyde overnight at 4 °C and embedded in paraplast. Serial sections were cut at 5 μm using a microtome, mounted on glass slides and rehydrated according to the standard protocols. Mounted slides were pretreated with a citrate buffer, pH 6.0, in a Black & Decker (Hampstead, MD, USA) steamer for 30 min, followed by a 10-min cool down. We used the following primary antibodies: anti-tau pThr231 (Millipore; AB9668; 1:200), anti-phospho-PHF-tau pSer202/Thr205 monoclonal antibody (Thermo Scientific; Clone AT8; MN1020, 1:200), anti-caspase-cleaved tau antibody (Invitrogen; AHB0061; 1:200) and anti-conformation-sensitive tau antibody (Clone MC1, gift of Dr. Peter Davies, Yeshiva University, Bronx, New York, USA, 1:200). Standard 2-day-immunostaining procedures with peroxidase-labelled streptavidin and DAB chromagen were carried out using a Vectastain Elite kit (Vector Laboratories; PK-6100). Hematoxylin counterstaining was used to provide cytological detail. Images were obtained using an inverted microscope (DMI6000B, Leica Microsystems Inc., Buffalo Grove, IL, USA). The number of p-tau (Thr231)-positive neurons and AT8-positive neurons was determined using the Image J software with colour deconvolution plug-in and Cell Counter analysis tools (NIH). Aβ40- and Aβ42-specific ELISA Cortex and hippocampus were dissected and homogenized in ice-cold guanidine buffer (5 M guanidine hydrochloride/50 mM TrisCl, pH 8.0). Aβ40 and Aβ42 levels were determined in samples using human-specific ELISA kits (Invitrogen) according to the manufacturer’s instructions. For human Aβ40 and Aβ42 ELISA, a monoclonal antibody specific against the N-terminus of human Aβ was used as the capturing antibody and a rabbit antibody specific for the C-terminus of either Aβ40 or Aβ42 was used as the detecting antibody [21] . For mouse Aβ40-specific sandwich ELISA, the capturing and biotinylated detecting antibodies were monoclonal anti-mouse Aβ raised against amino-acid residues 1–20 (Invitrogen, AMB0062) and rabbit polyclonal anti-Aβ40 biotin conjugate (Invitrogen), respectively [38] , [39] . For mouse Aβ42-specific sandwich ELISA, the capturing and detecting antibodies were AMB0062 and rabbit polyclonal anti-Aβ42 biotin conjugate (Invitrogen), respectively [38] , [39] . Synthetic mouse Aβ40 and Aβ42 (American Peptide Co., Sunnyvale, CA, USA) were used as standards. The lower detection limits for these ELISA assays are 0.5 pmol g −1 of Aβ40 and Aβ42, as reported [38] , [39] . Western blotting All samples were lysed in RIPA buffer (50 mM Tris, pH 8.0, 150 mM NaCl, 0.1% SDS, 1.0% NP-40, 0.5% sodium deoxycholate and Roche Applied Science, Indianapolis, IN, USA, protease inhibitor cocktail). Samples were then subjected to SDS–PAGE gel electrophoresis and transferred to a nitrocellulose membrane. Membranes were blocked with 5% milk, incubated with primary antibody and then incubated with the appropriate horse radish peroxidase-conjugated secondary antibody. Membranes were then treated with Immobilon Western ECL detection buffers (Millipore), exposed to CL-XPosure film (Thermo Scientific) and developed in a X-OMAT 3000 RA film processor (Kodak, Rochester, NY, USA). The following antibodies were used: anti-tau phospho Threonine 231, Millipore), anti-LRP-85 (Abcam), anti-RAGE (Santa Cruz Biotechnology Inc.), anti-neprilysin (R&D Systems), anti-IDE (Millipore, AB9210), anti-APP (Millipore) and horse radish peroxidase-conjugated goat anti-mouse IgG (Bio-Rad). Full scans of western blots are provided in Supplementary Fig. S5 . Measurement of sAPP-β levels and β-secretase activity sAPP-β levels in the brain of APP sw/0 Pdgfrβ +/+ and APP sw/0 Pdgfrβ +/− mice were measured using the ELISA kit (Covance) [39] and β-secretase activity was determined using a β-secretase activity kit (Abcam). In vivo microdialysis and ISF Aβ half-life determination In vivo microdialysis was used to measure soluble Aβ40 and Aβ42 steady-state levels in the hippocampus of awake, freely moving 3- to 4-month-old APP sw/0 Pdgfrβ +/+ and APP sw/0 Pdgfrβ +/− mice. Under isoflurane anesthetic, an intracerebral guide cannula MRB-5 (Bioanalytical Systems, West Lafayette, IN, USA) was stereotaxically implanted into the left hippocampus of the mouse (coordinates: AP −3.1 mm, L +2.4 mm and DV −0.6 mm at a 12° angle). A small head block (Instech laboratories, Plymouth Meeting, PA, USA) that provides tether anchoring to the freely moving system was attached to the skull. The cannula and the head block were cemented into place using dental acrylic. The microdialysis probes had a 2-mm, 38-kDa molecular weight cutoff membrane (Bioanalytical Systems) and were washed with 4% bovine serum albumin -artificial cerebrospinal fluid (aCSF) (Harvard Apparatus, Holliston, MA, USA) before use. After implantation of the guide cannula, the stylet was removed and the microdialysis probe inserted through the guide cannula into the hippocampus. The tethering system connected to a swivel (Instech) and counter balance arm (Instech) allowed unrestricted movement of the animal. The mice were allowed to recover from anesthesia and were housed in the freely moving system with ad libitum access to food and water throughout the experiment. The inlet tract of the microdialysis probe was connected to a PHD 2000 programmable syringe pump (Harvard Apparatus) using FEP tubing (SciPro, Sanborn, NY, USA), and 4% bovine serum albumin-aCSF was perfused continuously at a flow rate of 1 μl min −1 . Microdialysates were collected every 60 min into polypropylene tubes in a refrigerated fraction collector (Havard Apparatus). A stable baseline ISF Aβ40 and Aβ42 concentrations were obtained within 4 h followed by an intraperitoneal injection of Compound E (20 mg kg −1 , Millipore) [25] . In order to measure the elimination half-life ( t 1/2 ) of Aβ40 and Aβ42, eight additional 1-h microdialysates were collected. The t 1/2 of Aβ was calculated in the GraphPad Prism 5.0 software using the slope (k′) of the linear regression that included all fractions between drug delivery and when Aβ concentrations plateau ( t 1/2 =0.693/k, where k=2.303k′) [40] . The mice were perfused at the end of the experiment and probe-placement was verified. Measurements of soluble human Aβ40 and Aβ42 levels were performed using ELISA as described above. CY3-Aβ40 uptake and internalization by pericytes To isolate brain murine pericytes, isolated microvessel fragments from mouse cortex and hippocampus were digested for 12 h at 37 °C with collagenase A (Roche Applied Science), followed by constant shaking and vigorous pipetting every 3–4 h (ref. 6 ). The cells were then spun down and washed with PBS and plated in a complete medium containing Dulbecco’s Modified Eagle Medium (DMEM), 10% fetal bovine serum, 1% non-essential amino acids, 1% vitamins and 1% antibiotic/antimycotic on plastic (non-coated) tissue culture plates. After 6–12 h, the non-adherent cells were rinsed away and fresh medium was replaced every 2–3 days. Cultures were confirmed to be morphologically consistent with pericyte cultures and were PDGFRβ-positive, desmin-positive, glial fibrillar acidic protein-negative, aquaporin 4-negative, microtubule-associated protein 2-negative, NeuN-negative, von Willebrand Factor-negative and ionized calcium-binding adapter molecule 1-negative. Primary pericytes were plated into an eight-well chambered coverglass (Nunc, Thermo Scientific) and grown overnight. For Cy3-Aβ40 uptake experiments, pericytes were initially incubated with 1 μM Cy3-Aβ40 in DMEM at 4 °C for 1 h. Unbound Cy3-Aβ40 was removed by several washes with cold DMEM. Cy3-Aβ40 uptake was determined at 37 °C after 30 min incubation with and without 50 μg ml −1 non-immune IgG or specific function-blocking antibodies raised against the extracellular domain of LRP1 (Santa Cruz Biotechnology; sc-16166), LRP2 (a generous gift from Dr Scott Argraves, Medical University of South Carolina), very low-density lipoprotein receptor (R&D Systems; AF2258) and low-density lipoprotein receptor (R&D Systems; AF2255) [6] . Cy3-Aβ40 (1 μM) internalization and lysosomal colocalization in pericytes were determined 48 h after siRNA silencing of Lrp1, Lrp2 , Vldlr , Ldlr , Apoer2 or control siRNA (si Ctrl ) [6] . Adenoviral-mediated re-expression of the LRP1 minigene (Ad.m LRP1 ) or GFP was performed in pericytes with silenced Lrp1 . LysoTracker green DND-26 (Invitrogen) was added at 100 nM and incubated for 30 min at the end of the experiment. Cells were then fixed with 4% paraformaldehyde (PFA), washed with PBS, briefly incubated with 0.1% Triton X-100 for 20 s and then stained with Alexa Fluor phalloidin conjugates, F-actin (Invitrogen) and Hoechst 33342 (Invitrogen). Slides were scanned using Zeiss 510 confocal microscope (Carl Zeiss MicroImaging Inc., Thornwood, NY, USA). The Cy3-Aβ40 relative intensity and its lysosomal colocalization in pericytes were measured with the NIH Image J software. Cell death in Aβ-treated pericyte cultures Brain murine pericytes were plated into an eight-well chambered coverglass (Nunc, Thermo Scientific). Cells were cultured for 7 days in the presence and absence of 5 μM Aβ40. Medium with and without 5 μM Aβ40 was replaced after 3 days. Cell viability was quantified using a fluorescent Live/Dead Viability/Cytotoxicity kit according to the manufacturer’s instruction (Invitrogen). In some experiments, cells were treated with anti-LRP1 antibody or si Lrp1 for 7 days, as described above. Images were obtained using an inverted microscope (DMI6000B, Leica Microsystems Inc., Buffalo Grove, IL, USA). Data were analysed with the NIH ImageJ counter tool. Behavioural testing For the novel object recognition test [41] , [42] , mice were acclimatized to a 25-cm 3 cubic box for 10 min, and then exposed at three-time-point trials to two objects affixed to the floor, equidistant to the two nearest walls. Mice were placed in a corner equidistant to both objects, minimizing spatial memory confounds. Starting position for mice was rotated, and objects counterbalanced throughout the test. All trials were videotaped for 5 min. Baseline trial was performed 24 h after acclimatization with two identical objects. A choice trial was performed 90 min after baseline, replacing one familiar object with a novel object and keeping one baseline object constant. Total duration of exploratory approaches to familiar or novel objects was measured and was defined as sniffing or touching an object with the snout at a critical distance of <1 cm from object. The novelty exploration index was calculated as time spent exploring the novel object over total time exploring both objects. To assess burrowing behaviour, mice were individually placed in rat cages equipped with a burrow made from a 200-mm long and 70-mm-diameter tube of polyvinyl chloride (PVC) plastic [43] . One end of the tube was closed by a PVC cap. The open end of the tube was raised ~30 mm by drilling in two supporting screws [44] . The burrow was filled with 200 g of mouse food pellets, and the mice were allowed to burrow for 3 h. The weight of the remaining food pellets inside the burrow was determined to obtain a measurement of the amount burrowed. For the younger age group (1-month old), a PVC tube of 50 mm in diameter and 250 g of mouse food were used instead. All other procedures were performed identically to the older mouse groups. To assess nest construction behaviour, mice were individually placed in their home cages with a preweighed nestlet ~1 h before the dark phase. The nests were assessed the next morning and given a score of 1–5 based on the nest construction score [41] . Any unused nestlet was weighed to determine the percentage of nestlet used. Voltage-sensitive dye imaging of cortical activity For VSD imaging [6] , a cranial window was placed over the somatosensory cortex using the same procedure as for Multiphoton imaging above. After removing the dura, without causing any cranial bleeding, RH-1692 VSD (Optical Imaging), dissolved in aCSF was applied to the exposed cortex. The brain was washed with aCSF for 5 min, covered with low-melt agarose dissolved in aCSF (~1.3%), sealed with a coverslip and the skull was secured to a custom-built microscopy frame. Images were collected using a Pixelfly CCD camera coupled to the CamWare 3.0 software. RH-1692 was excited using a 627-nm LED light source and imaged using a custom-built Olympus 2 × epifluorescent microscope. Images were collected for 500 ms before and after a mechanical deflection of the hindlimb 5 ms in duration. The responses were averaged from 10–20 trials per animal. Stimulation trial signals were divided by baseline signal profiles collected in the absence of stimulation. The signal intensity was quantified by placing a circular region area of interest over the hindlimb region using the NIH Image software. The change in fluorescent intensity (ΔF/F 0 ) was calculated as a percent change by dividing the signal intensity change after stimulation (ΔF) by the average intensity taken before stimulation (F 0 ) [6] . The time-lapse ΔF/F 0 profiles of VSD signal responses were plotted using ImageJ. The peak amplitude and time-to-peak in fluorescent VSD signal in the hindlimb somatosensory cortex after stimulation were taken from readings of generated VSD time-lapse profiles [6] . Laser doppler flowmetry Cerebral blood flow responses to vibrissal stimulation in anesthetized 3- to 4-month-old APP sw/0 Pdgfrβ +/+ and APP sw/0 Pdgfrβ +/− mice (750 mg kg −1 urethane and 50 mg kg −1 chloralose) were determined with laser Doppler flowmetry [5] , [21] . The tip of the laser Doppler probe (Transonic Systems Inc., Ithaca, NY, USA) was stereotaxically placed 0.5 mm above the dura of the cranial window. The right vibrissae was cut to about 5 mm and stimulated by gentle stroking at 3–4 Hz for 1 min with a cotton-tip applicator. The percentage increase in cerebral blood flow (CBF) because of vibrissal stimulation was obtained from the baseline CBF and stable maximum plateau and was averaged for the three trials. Arterial blood pressure was monitored continuously during the experiment. pH and blood gases were monitored before and after CBF recordings. No significant changes in these physiological parameters were found between different genotypes and ages. Statistical analysis Sample sizes were calculated using nQUERY assuming a two-sided alpha-level of 0.05, 80% power and homogeneous variances for the two samples to be compared, with the means and common s.d. for different parameters predicted from published data and our previous studies. All animals were included in the study. F-test was conducted to ensure that the data meet the assumptions of the tests. The variance was similar between the groups that are statistically compared. Data were analysed using Student’s t -test or using multifactorial analysis of variance followed by Tukey’s post-hoc tests. A P -value <0.05 was considered statistically significant in all studies. How to cite this article: Sagare, A. P. et al . Pericyte loss influences Alzheimer-like neurodegeneration in mice. Nat. Commun. 4:2932 doi: 10.1038/ncomms3932 (2013).